Pigment cell interactions and differential xanthophore recruitment underlying zebrafish stripe reiteration andDaniopattern evolution Fishes have diverse pigment patterns, yet mechanisms of pattern evolution remain poorly understood. In zebrafish, Danio rerio , pigment–cell autonomous interactions generate dark stripes of melanophores that alternate with light interstripes of xanthophores and iridophores. Here, we identify mechanisms underlying the evolution of a uniform pattern in D. albolineatus in which all three pigment cell classes are intermingled. We show that in this species xanthophores differentiate precociously over a wider area, and that cis regulatory evolution has increased expression of xanthogenic Colony Stimulating Factor-1 (Csf1). Expressing Csf1 similarly in D. rerio has cascading effects, driving the intermingling of all three pigment cell classes and resulting in the loss of stripes, as in D. albolineatus . Our results identify novel mechanisms of pattern development and illustrate how pattern diversity can be generated when a core network of pigment–cell autonomous interactions is coupled with changes in pigment cell differentiation. Among vertebrates, teleost fishes have some of the most striking and diverse adult pigment patterns and these patterns can have important roles in behaviour and speciation [1] , [2] , [3] , [4] , [5] , [6] , [7] , [8] . Although mechanisms of pattern formation are starting to be elucidated, we still know very little about the genetic and cellular bases of pattern diversification. Fishes in the genus Danio can potentially shed light on pattern evolution because of their diversity of patterns [9] , [10] , [11] , [12] , [13] , and the phylogenetic proximity of these species to zebrafish D. rerio [14] , in which pattern development is being studied intensively. In zebrafish, dark stripes, comprising melanophores and a few iridescent iridophores, alternate with light interstripes of yellow-orange xanthophores and abundant iridophores, all of which are located in the hypodermis, between the skin and myotome [15] , [16] , [17] , [18] . This striped pattern arises through interactions between pigment cells and their environment, as well as interactions within and between pigment cell classes [19] , [20] , [21] , [22] , [23] , [24] , [25] , [26] ; remarkably, the dynamics of some of these interactions resemble those predicted by Turing models of pattern formation [27] , [28] , [29] . Within Danio a pattern that includes horizontal stripes and interstripes at some stage of post-embryonic development is likely to be ancestral [10] , [30] , [31] . These stripes and interstripes persist and can be reiterated in the adults of some species, and are most distinctive in D. rerio ( Fig. 1a ); similarly organized, albeit fewer, stripes and interstripes are found in the close zebrafish relative, spotted danio, D. nigrofasciatus . At the opposite end of a stripe continuum [6] is the pearl danio, D. albolineatus , and very closely related species or subspecies (for example, D. roseus ), in which pigment cells of different classes are intermingled and nearly uniformly distributed, and only a residual interstripe remains ( Fig. 1a ). Although ambiguities in species relationships [14] , [32] , [33] , [34] preclude assessing the polarity of some evolutionary transformations in Danio , developmental and genetic analyses indicate that an ancestral pattern of stripes and interstripes has been elaborated upon in D. rerio and obscured in D. albolineatus [9] , [10] , [31] , [35] , suggesting that further analyses of these divergent phenotypes could inform our understanding of pattern evolution more generally. 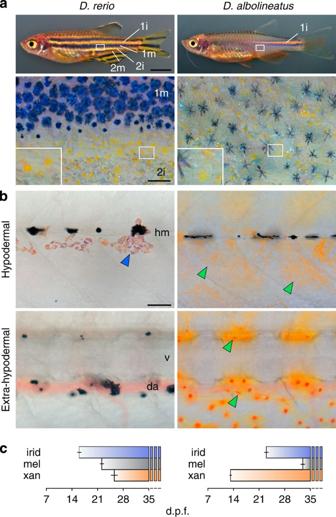Figure 1: Different pigment patterns ofD. rerioandD. albolineatus. (a)D. reriohave interstripes with intervening stripes. The primary interstripe (1i) is first to develop, followed by primary stripes of melanophores (1 m) and secondary interstripes (2i) and stripes (2 m)42. Xanthophores (lower, inset) and melanophores are segregated spatially.D. albolineatusdevelop only a single incomplete interstripe, and melanophores and xanthophores are intermingled across the flank. (b) Early in adult pigment pattern development inD. rerio(stage AR ref.42), xanthophores had not yet differentiated and only adult iridophores (blue arrowhead) and residual early larval melanophores were observed hypodermally. At the same stage inD. albolineatus, numerous xanthophores (green arrowheads) had differentiated hypodermally and extra-hypodermally. hm, horizontal myoseptum; v, vertebral column; da, dorsal aorta. (c) In comparison withD. rerio, xanthophores ofD. albolineatusdeveloped precociously. Shown are mean±s.e.m. days post fertilization when pigment cells of each class first appeared (species difference across all classes,F2,18=158,P<0.001;n=5D. rerio;n=3D. albolineatus). Scale bars, 1 mm (aupper); 200 μm (alower); 60 μm (b). Figure 1: Different pigment patterns of D. rerio and D. albolineatus . ( a ) D. rerio have interstripes with intervening stripes. The primary interstripe (1i) is first to develop, followed by primary stripes of melanophores (1 m) and secondary interstripes (2i) and stripes (2 m) [42] . Xanthophores (lower, inset) and melanophores are segregated spatially. D. albolineatus develop only a single incomplete interstripe, and melanophores and xanthophores are intermingled across the flank. ( b ) Early in adult pigment pattern development in D. rerio (stage AR ref. 42 ), xanthophores had not yet differentiated and only adult iridophores (blue arrowhead) and residual early larval melanophores were observed hypodermally. At the same stage in D. albolineatus , numerous xanthophores (green arrowheads) had differentiated hypodermally and extra-hypodermally. hm, horizontal myoseptum; v, vertebral column; da, dorsal aorta. ( c ) In comparison with D. rerio , xanthophores of D. albolineatus developed precociously. Shown are mean±s.e.m. days post fertilization when pigment cells of each class first appeared (species difference across all classes, F 2,18 =158, P <0.001; n =5 D. rerio ; n =3 D. albolineatus ). Scale bars, 1 mm ( a upper); 200 μm ( a lower); 60 μm ( b ). Full size image In this report, we investigated the mechanisms responsible for the nearly uniform pattern of D. albolineatus as compared with the reiterated stripes and interstripes of D. rerio. Besides the overall pattern, these species differ strikingly in xanthophore abundance, with many more of these cells present in D. albolineatus hypodermally, and also ‘extra-hypodermally’ in more medial locations ( Fig. 1b ). Although xanthophores of D. rerio require thyroid hormone (TH), many xanthophores of D. albolineatus develop independently of TH, suggesting the evolution of a compensatory factor in this species [26] . Here we show that a precocious, widespread differentiation of xanthophores in D. albolineatus is associated with increased expression of a xanthogenic factor, colony-stimulating factor 1 (Csf1), resulting in part from cis regulatory evolution at the csf1a locus. When Csf1 is expressed correspondingly in D. rerio , pigment cells are intermingled and a uniform pattern largely recapitulating that of D. albolineatus developed, owing to a xanthophore-dependent repression of iridophore organization and concomitant failure of stripe–interstripe boundary formation. Finally, we show that interstripe iridophores in D. rerio not only specify melanophore stripe orientation and position [22] , [23] , but also determine stripe width, and that development of these cells has been markedly curtailed in D. albolineatus . Our results identify molecular and cellular changes contributing to a uniform pattern in D. albolineatus and illustrate how changes in the time and place of pigment cell differentiation have cascading effects on pattern formation. More xanthophores and increased Csf1 in D. albolineatus Analyses of developing larvae revealed that xanthophores are the first adult pigment cells to differentiate in D. albolineatus , but the last to differentiate in D. rerio ( Fig. 1b,c ; Supplementary Fig. 1 ). We hypothesized that precocious development of especially abundant xanthophores in D. albolineatus evolved through changes in the expression of Csf1. In D. rerio , Csf1 signalling through the Csf1 receptor (Csf1r) [36] , [37] is essential for xanthophore differentiation, proliferation and survival [19] , [20] , [38] . Csf1 is expressed by interstripe iridophores and promotes the development of interstripe xanthophores; this factor is also expressed in the skin and its ectopic expression drives ectopic xanthophore development [22] . Moreover, analyses of D. rerio × D. albolineatus hybrid phenotypes have suggested evolutionary changes in the Csf1 pathway [9] , [31] . By reverse transcriptase (RT)-PCR of both species, we found that the two Csf1 loci, csf1a and csf1b , were expressed in skin and iridophores ( Supplementary Fig. 2a ). By quantitative RT-PCR of ‘internal’ tissue denuded of skin, but including cells adjacent to hypodermis, csf1a and csf1b transcript abundances were elevated by as much as four- to sixfold in D. albolineatus from early stages ( Fig. 2a ; Supplementary Fig. 2b ). Thus, xanthogenic Csf1 is upregulated when xanthophores first develop in D. albolineatus , particularly internally where extra-hypodermal xanthophores arise, and adjacent to where hypodermal xanthophores develop. 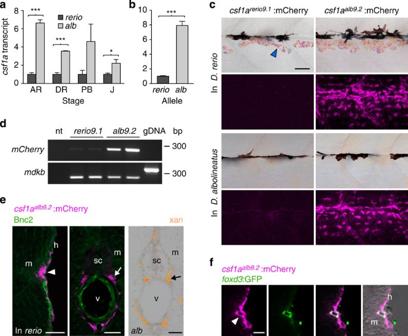Figure 2: Enhanced Csf1 expression inD. albolineatusthroughcisregulatory evolution. (a)csf1atranscript abundance during adult pigment pattern development inD. albolineatusrelative toD. reriofor internal trunk tissue (mean±s.e.m.;n=3 biological replicates for all samples). ***P<0.0001; *P<0.05. (Stages: AR, anal fin ray appearance; DR, dorsal fin ray appearance; PB, pelvic bud appearance; J, juvenile.) (b) Increased expression ofD. albolineatus csf1aallele inD. rerio×D. albolineatushybrids (mean±s.e.m.; pairedt=12.8, d.f.=4,P<0.0005;n=5 biological replicates). (c) mCherry in AR+ stageTg(csf1arerio9.1:mCherry)(left) andTg(csf1aalb9.2:mCherry)(right), inD. rerio(top) andD. albolineatus(bottom). Images forcsf1arerio9.1:mCherrywere exposed twice as long yet show only background fluorescence. (d)csf1arerio9.1:mCherrywas detectable at low levels.midkine b(mdkb), control target amplifying 259 bp from cDNA or 334 bp with intron from genomic DNA (gDNA); nt, no template. (e)csf1aalb9.2:mCherry inD. rerio(magenta, arrowhead) in hypodermis (h), adjacent to the myotome (m) and also medially (arrow) in the vicinity of the spinal cord (sc) and vertebral column (v), corresponding to ventral motor nerves. Basonuclin-2 (Bnc2; green) promotes Csf1 expression inD. rerio22, but Bnc2+cells did not co-express mCherry. Right, extra-hypodermal xanthophores (arrow) inD. albolineatus. (f) At the hypodermis,csf1aalb9.2:mCherry was expressed by Foxd3+glia (green) of the lateral line nerve (arrow) and other cells. Scale bars, 40 μm (c,eleft 2 panels,f), 60 μm (eright 2 panels). Figure 2: Enhanced Csf1 expression in D. albolineatus through cis regulatory evolution. ( a ) csf1a transcript abundance during adult pigment pattern development in D. albolineatus relative to D. rerio for internal trunk tissue (mean±s.e.m. ; n =3 biological replicates for all samples). *** P <0.0001; * P <0.05. (Stages: AR, anal fin ray appearance; DR, dorsal fin ray appearance; PB, pelvic bud appearance; J, juvenile.) ( b ) Increased expression of D. albolineatus csf1a allele in D. rerio × D. albolineatus hybrids (mean±s.e.m. ; paired t =12.8, d.f.=4, P <0.0005; n =5 biological replicates). ( c ) mCherry in AR+ stage Tg(csf1a rerio9.1 :mCherry) (left) and Tg(csf1a alb9.2 :mCherry) (right), in D. rerio (top) and D. albolineatus (bottom). Images for csf1a rerio9.1 :mCherry were exposed twice as long yet show only background fluorescence. ( d ) csf1a rerio9.1 :mCherry was detectable at low levels. midkine b ( mdkb ), control target amplifying 259 bp from cDNA or 334 bp with intron from genomic DNA (gDNA); nt, no template. ( e ) csf1a alb9.2 :mCherry in D. rerio (magenta, arrowhead) in hypodermis (h), adjacent to the myotome (m) and also medially (arrow) in the vicinity of the spinal cord (sc) and vertebral column (v), corresponding to ventral motor nerves. Basonuclin-2 (Bnc2; green) promotes Csf1 expression in D. rerio [22] , but Bnc2 + cells did not co-express mCherry. Right, extra-hypodermal xanthophores (arrow) in D. albolineatus . ( f ) At the hypodermis, csf1a alb9.2 :mCherry was expressed by Foxd3 + glia (green) of the lateral line nerve (arrow) and other cells. Scale bars, 40 μm ( c , e left 2 panels, f ), 60 μm ( e right 2 panels). Full size image cis regulatory evolution underlying csf1a expression To understand the mechanism underlying evolutionary change in Csf1 expression, we focused on csf1a , for which the species difference lasts into late stages. To test for cis regulatory change at the csf1a locus, we crossed D. albolineatus to D. rerio and assayed species-specific transcript abundance in the averaged trans regulatory background of the hybrid. If differences are in cis , the D. albolineatus allele should be expressed higher than the D. rerio allele; if differences are in trans , alleles should be expressed similarly. These analyses revealed eightfold higher expression of the D. albolineatus csf1a allele, strongly suggesting that cis regulatory changes contribute to the differential expression between species ( Fig. 2b ). To further test for cis regulatory evolution, we cloned ~9-kb regions between a conserved distal sequence and the csf1a translational start sites. We used these fragments, csf1a rerio9.1 and csf1a alb9.2 , to drive mCherry in multiple stable transgenic lines in each species. Each of the nine lines for csf1a rerio9.1 :mCherry failed to express mCherry at levels visualizable by native fluorescence or immunohistochemistry, although low levels of transcript were detectable by RT-PCR ( Fig. 2c,d ). By contrast, each of the six lines for csf1a alb9.2 :mCherry exhibited robust expression from early larval stages. Similar to native csf1a transcript in D. rerio [22] , csf1a alb9.2 :mCherry was expressed in the hypodermis. csf1a alb9.2 :mCherry also was expressed medially in peripheral nerves, adjacent to where extra-hypodermal xanthophores develop in D. albolineatus ( Fig. 2e ) and where xanthophore precursors occur in D. rerio [26] ; extra-hypodermal csf1a transcript has not been detectable by in situ hybridization in D. rerio [22] . Finally, csf1a alb9.2 :mCherry was expressed by Foxd3 + glia of the lateral line ( Fig. 2f ) and in several other tissues as well ( Supplementary Fig. 3 ). Alignments of csf1a rerio9.1 and csf1a alb9.2 revealed conserved regions missing or disrupted in D. albolineatus ( Supplementary Fig. 3a ), suggesting that increased expression may have resulted from the loss of one or more repressor elements. As an initial test of this possibility, we focused on an altered proximal region, where repressors often are found [39] , [40] , and generated transgenic reporter lines for deletions of corresponding regions in D. rerio . In contrast to lines for csf1a rerio9.1 , in which mCherry was never detectable, deletion lines exhibited high mCherry expression from early stages that overlapped with sites of csf1a alb9.2 expression, yet specific domains varied markedly across constructs and replicates ( Supplementary Fig. 3b ), suggesting a derepression but also dysregulation subject to integration site effects. Although additional regulatory changes are presumed, these findings support a model in which loss of one or more repressor elements contributed to earlier, higher and more widespread expression of csf1a in D. albolineatus , contributing to earlier, more numerous and more broadly distributed xanthophores. Csf1 recruits extra xanthophores and drives stripe loss We next asked whether changes in the time and place of xanthophore differentiation could account for the more uniform pattern of D. albolineatus . We reasoned that xanthophores, as the first adult pigment cells to appear in D. albolineatus ( Fig. 1b,c ), might have a critical role in specifying pattern, much as iridophores, the first adult pigment cell to appear in D. rerio , specify the location and orientation of the first stripes and interstripe [22] , [23] . To test this possibility, we used the ubiquitous, heat-shock inducible promoter of hsp70l to overexpress Csf1a and thereby generated extra xanthophores in D. rerio , beginning when differences in Csf1 expression were first detectable between species. The resulting pattern resembled that of D. albolineatus , with (ectopic) extra-hypodermal xanthophores, supernumerary hypodermal xanthophores and stripes of intermingled melanophores and xanthophores that extended to the ventral margin of the flank ( Fig. 3a,c,d,l,m ; Supplementary Fig. 4a ). These fish also had extra melanophores, likely reflecting an indirect effect of Csf1 mediated through xanthophores, which provide trophic support to melanophores [19] , [28] , [41] ( Supplementary Fig. 4b ). 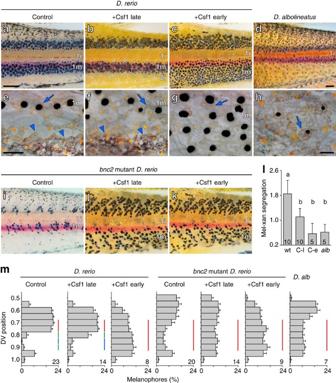Figure 3: Time and pattern of xanthophore differentiation is critical for pattern outcome. (a–d) When Csf1 was induced and extra xanthophores developed early inD. rerio(c; stage AR+ ref.42), stripes extended to the ventral margin of the flank, and secondary interstripes failed to develop similar toD. albolineatus(d). When induced late (b; SA+), stripe widths were similar to controls (a). (e–h) Higher-magnification images showing organized, interstripe iridophores (arrowheads ineandf) or their absence (g,h); scattered iridophores (arrows) are present in all panels. Yellow-orange xanthophores were segregated from melanophores ine, but intermingled with melanophores inf–h. (i–k)bnc2mutants fail to develop secondary interstripe iridophores and Csf1 overexpression either early or late resulted in a uniform pattern. (l) Melanophore–xanthophore segregation was less in Csf1-overexpressingD. rerioandD. albolineatus(‘wt,’ non-transgenic siblings heat shocked similarly) regardless of stripe presence (‘C-l,’ Csf1 late overexpression) or absence (‘C-e,’ Csf1 early overexpression;alb,D. albolineatus). Common letters above bars indicate groups not significantly different (P>0.05) in Tukey Kramerpost hoccomparisons; overallF3,27=9.2,P<0.0005). Shown are means±s.e.m.; sample sizes are indicated within each bar. (m) Melanophore frequencies at dorsal–ventral positions on the ventral flank (0.5=horizontal myoseptum, 1=ventral margin of myotomes). Vertical bars of the same colour indicate positions not significantly different in Tukey Kramerpost hoccomparisons (P>0.05): a distinct discontinuity in melanophore distribution, representing the stripe–interstripe boundary, was evident in control and Csf1-late-overexpressingD. reriobut not other backgrounds. For clarity only comparisons across positions 0.7–0.9 are shown. Shown are means±s.e.m.; sample sizes are indicated at the lower right of each plot. Scale bars, 400 μm (a, fora–candi–k), 400 μm (d); 60 μm (efore–g); 60 μm (h). Figure 3: Time and pattern of xanthophore differentiation is critical for pattern outcome. ( a – d ) When Csf1 was induced and extra xanthophores developed early in D. rerio ( c ; stage AR+ ref. 42 ), stripes extended to the ventral margin of the flank, and secondary interstripes failed to develop similar to D. albolineatus ( d ). When induced late ( b ; SA+), stripe widths were similar to controls ( a ). ( e – h ) Higher-magnification images showing organized, interstripe iridophores (arrowheads in e and f ) or their absence ( g , h ); scattered iridophores (arrows) are present in all panels. Yellow-orange xanthophores were segregated from melanophores in e , but intermingled with melanophores in f – h . ( i – k ) bnc2 mutants fail to develop secondary interstripe iridophores and Csf1 overexpression either early or late resulted in a uniform pattern. ( l ) Melanophore–xanthophore segregation was less in Csf1-overexpressing D. rerio and D. albolineatus (‘wt,’ non-transgenic siblings heat shocked similarly) regardless of stripe presence (‘C-l,’ Csf1 late overexpression) or absence (‘C-e,’ Csf1 early overexpression; alb , D. albolineatus ). Common letters above bars indicate groups not significantly different ( P >0.05) in Tukey Kramer post hoc comparisons; overall F 3,27 =9.2, P <0.0005). Shown are means±s.e.m. ; sample sizes are indicated within each bar. ( m ) Melanophore frequencies at dorsal–ventral positions on the ventral flank (0.5=horizontal myoseptum, 1=ventral margin of myotomes). Vertical bars of the same colour indicate positions not significantly different in Tukey Kramer post hoc comparisons ( P >0.05): a distinct discontinuity in melanophore distribution, representing the stripe–interstripe boundary, was evident in control and Csf1-late-overexpressing D. rerio but not other backgrounds. For clarity only comparisons across positions 0.7–0.9 are shown. Shown are means±s.e.m. ; sample sizes are indicated at the lower right of each plot. Scale bars, 400 μm ( a , for a – c and i – k ), 400 μm ( d ); 60 μm ( e for e – g ); 60 μm ( h ). Full size image Xanthophores can repress interstripe development Besides alterations in melanophore and xanthophore distributions, D. rerio overexpressing Csf1 from early stages had changes to iridophore patterning. D. rerio normally develop a single ‘primary’ interstripe of iridophores followed by two primary stripes of melanophores above and below. Later, ‘secondary’ interstripes are added further dorsally and ventrally, followed by secondary stripes [42] . In Csf1-overexpressing D. rerio , however, iridophores were fewer and aggregations of secondary interstripe iridophores failed to develop, similar to D. albolineatus ( Fig. 3e,g,h ). Because changes in iridophore pattern could have resulted from Csf1-dependent increases in either xanthophores or melanophores, we used a transgenic line [22] for melanogenic Kit ligand-a [43] , [44] to generate extra melanophores, but not xanthophores, at the same stages: in these fish iridophores were distributed similarly to the wild type ( Supplementary Fig. 5 ). Together these findings indicate that overexpression of Csf1 and xanthophore population expansion can repress iridophore organization, despite the normal role of iridophores in promoting xanthophore development [22] . This suggests that changes in differentiation timing and location can have cascading effects, markedly altering the pattern even without changes in the network architecture of pigment–cell autonomous interactions [19] , [20] , [22] , [23] , [27] , [28] . To assess the limits of such pattern plasticity, we overexpressed Csf1 in D. rerio at a later stage, when secondary interstripe iridophores had started to develop already. In these fish, supernumerary xanthophores were intermingled with melanophores, yet the secondary interstripe persisted and melanophores were confined to the normal domain of the ventral primary stripe ( Fig. 3b,f,l,m ), suggesting that once a secondary interstripe has been established it is resistant to Csf1-dependent xanthophore repression. To further test that persistence of a stripe–secondary interstripe boundary in late Csf1-overexpressing fish depended on iridophores, we repeated these experiments in bnc2 mutant D. rerio , which have severe deficiencies in all three pigment cell classes and fail to form secondary interstripes [22] , [45] . In this background, Csf1 overexpression resulted in intermingled melanophores and xanthophores that extended to the margin of the flank, regardless of stage ( Fig. 3i–k,m ). Together these experiments suggest a ‘priority effect’ in which the first pigment cell class to differentiate in a given region can have a critical influence in specifying the pattern. Iridophores delimit stripe width To place these findings in an evolutionary context, we further examined iridophore development in both species, focusing on the ventral region of the flank ( Fig. 4a ). In D. rerio , iridophores initially populated the primary interstripe but were later found sparsely within the ventral primary stripe, and, subsequently, in aggregations further ventrally where they established a secondary interstripe. As iridophores increased in number, melanophores that had started to differentiate in the prospective secondary interstripe died or migrated away ( Fig. 4b ; Supplementary Movie 1 ). These observations suggested that iridophores not only initiate melanophore stripe patterning [22] , [23] but also terminate stripes once patterning has started. We tested this by ablating secondary interstripe iridophores using a transgene, pnp4a:nVenus-2a-nfnB , in which bacterial nitroreductase is expressed by the iridophore-specific promoter of purine nucleoside phosphorylase 4a , allowing targeted killing of iridophores by treatment with metronidazole [22] , [46] . In the absence of iridophores, melanophores persisted and the ventral primary melanophore stripe extended to the margin of the flank ( Fig. 4c ; Supplementary Fig. 6a–c ). 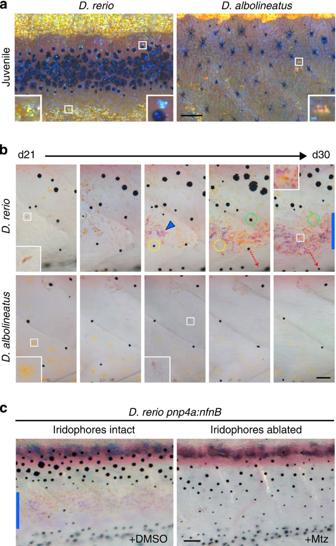Figure 4: Iridophore distributions and role in stripe termination. (a) JuvenileD. rerioandD. albolineatusimaged to highlight iridophores. ForD. rerio, insets show iridophores at the edge of the ventral secondary interstripe (left) and an iridophore in the stripe (right). ForD. albolineatus, inset shows one of only a few small aggregates of iridophores. (b) Development of ventral iridophores between 21 and 30 d.p.f. (stages PB+to SA). InD. rerio, iridophores (for example, inset, d21) were initially scattered among melanophores in the developing ventral primary melanophore stripe but subsequently formed aggregates (for example, arrowhead) at the site of the secondary ventral interstripe. Some melanophores initially in this region died; yellow and green dashed circles show initial positions for each of two melanophores and their absence on subsequent days. Other melanophores in this region translocated further dorsally or ventrally; dashed red arrow indicates one melanophore that moved ventrally). At day 30 (d30), inset shows first xanthophore to differentiate in the secondary interstripe and the vertical blue bar indicates overall interstripe width. InD. albolineatusat day 21 (d21), xanthophores are abundant (inset), but iridophores are scarce (for example, inset, middle panel) as are melanophores. (c) InD. rerio, ablation of ventral secondary interstripe iridophores by treatment with Mtz results in a failure of stripe termination. Blue bar, secondary interstripe in dimethyl sulfoxide (DMSO) control. Fish inbandcwere treated with epinephrine to contract pigment granules towards cell centres. Scale bars, 60 μm (a,b); 100 μm (c). Figure 4: Iridophore distributions and role in stripe termination. ( a ) Juvenile D. rerio and D. albolineatus imaged to highlight iridophores. For D. rerio , insets show iridophores at the edge of the ventral secondary interstripe (left) and an iridophore in the stripe (right). For D. albolineatus , inset shows one of only a few small aggregates of iridophores. ( b ) Development of ventral iridophores between 21 and 30 d.p.f. (stages PB+to SA). In D. rerio , iridophores (for example, inset, d21) were initially scattered among melanophores in the developing ventral primary melanophore stripe but subsequently formed aggregates (for example, arrowhead) at the site of the secondary ventral interstripe. Some melanophores initially in this region died; yellow and green dashed circles show initial positions for each of two melanophores and their absence on subsequent days. Other melanophores in this region translocated further dorsally or ventrally; dashed red arrow indicates one melanophore that moved ventrally). At day 30 (d30), inset shows first xanthophore to differentiate in the secondary interstripe and the vertical blue bar indicates overall interstripe width. In D. albolineatus at day 21 (d21), xanthophores are abundant (inset), but iridophores are scarce (for example, inset, middle panel) as are melanophores. ( c ) In D. rerio , ablation of ventral secondary interstripe iridophores by treatment with Mtz results in a failure of stripe termination. Blue bar, secondary interstripe in dimethyl sulfoxide (DMSO) control. Fish in b and c were treated with epinephrine to contract pigment granules towards cell centres. Scale bars, 60 μm ( a , b ); 100 μm ( c ). Full size image In D. albolineatus , iridophores were fewer initially and never formed ventral aggregations ( Fig. 4a,b ; Supplementary Movie 2 ) although in the adult these cells were scattered widely over the flank ( Supplementary Fig. 6d ). Thus, interstripe iridophores delimit the width of melanophore stripes in D. rerio , whereas development of these cells has been curtailed in D. albolineatus , a change that may itself be xanthophore-dependent (compare Fig. 3e,g,h ). Our results identify new interactions among pigment cell classes in D. rerio , elaborating upon a model for stripe development, and also suggest a new model for how evolutionary changes in pigment cell differentiation have contributed to the strikingly different pattern of D. albolineatus , and perhaps other species. Previous studies elucidated a complex network of interactions involving all three pigment cell classes in D. rerio ( Fig. 5a ) [19] , [20] , [21] , [22] , [23] , [24] , [25] , [26] , [27] , [28] . Iridophores promote the differentiation and localization of xanthophores at short range and repress their differentiation at long range. By producing extra pigment cells transgenically, we identified a reciprocal interaction in which xanthophores repress the development and organization of iridophores (interaction 1 in Fig. 5a ). A contribution of xanthophores to patterning iridophores during normal development is likewise suggested by defects in iridophore organization in xanthophore-deficient csf1r mutants [22] , [23] . Our analyses of phenotypes resulting from iridophore ablation further support the idea that iridophores influence melanophore distributions either directly or indirectly (interaction 2 in Fig. 5a ), presumably through a combination of short-range inhibition and longer-range attraction [22] , [23] . These experiments that either increased or decreased the numbers of pigment cells illustrate the critical role of cellular context in pattern formation: even with the core network of interactions unchanged, differences in the abundance and distribution of particular pigment cell classes can limit the sort of interactions in which cells participate, with consequences for the pattern that develops ( Fig. 5b ). 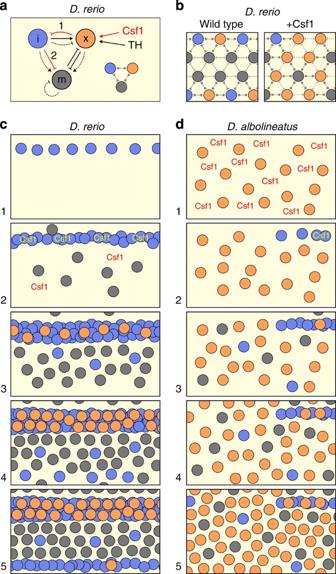Figure 5: Models for pattern formation and evolution. (a) Network of interactions among iridophores (i), xanthophores (x) and melanophores (m). Interactions are positive (→) or negative (); long-range interactions are indicated by dashed lines. Csf1 and TH both promote xanthophore development; Csf1 is also supplied by iridophores to xanthophores (i→x)22. When xanthophores are highly abundant, these cells can repress iridophore development (1). Iridophores attract melanophores (i→m), but also directly or indirectly repress melanophore survival and localization, and terminate stripe development (2). Simplified interaction diagram at lower right, corresponding tob. (b) When Csf1 is overexpressed inD. rerio, melanophores encounter more xanthophores and fewer iridophores, participate in only a subset of potential interactions and fail to receive positional information necessary to terminate primary stripes or initiate secondary stripes. Interactions between xanthophores are hypothetical. (c) Pattern development inD. rerio.(1) Iridophores differentiate at the horizontal myoseptum. (2) Melanophores arise dispersed over the flank while iridophores express Csf1, which is also expressed in the skin. (3) Locally high levels of Csf1 promote xanthophore differentiation in the interstripe as interactions involving all three classes of pigment cells refine the pattern of stripes and interstripes and additional iridophores infiltrate the stripe. (4) Iridophores begin to emerge beyond the stripe and initiate a secondary interstripe. (5) Iridophores of the secondary interstripe terminate the primary stripe, promote differentiation of secondary interstripe xanthophores and specify the location of secondary stripe development. Adult xanthophore precursors, and, later, incompletely differentiated xanthophores are distributed sparsely in stripes as well26,50(not shown). (d) Pattern development inD. albolineatus. (1) Initially high expression of iridophore-independent Csf1 promotes early, widespread xanthophore development. (2) A few iridophores develop near the horizontal myoseptum posteriorly. (3) Melanophores begin to appear scattered over the flank as do additional iridophores. (4–5) Residual stripes begin to form posteriorly around the residual interstripe35, but this pattern is obscured by widespread melanophores and xanthophores that ultimately fail to resolve into stripes and interstripes. Figure 5: Models for pattern formation and evolution. ( a ) Network of interactions among iridophores (i), xanthophores (x) and melanophores (m). Interactions are positive (→) or negative ( ); long-range interactions are indicated by dashed lines. Csf1 and TH both promote xanthophore development; Csf1 is also supplied by iridophores to xanthophores (i→x) [22] . When xanthophores are highly abundant, these cells can repress iridophore development (1). Iridophores attract melanophores (i→m), but also directly or indirectly repress melanophore survival and localization, and terminate stripe development (2). Simplified interaction diagram at lower right, corresponding to b . ( b ) When Csf1 is overexpressed in D. rerio , melanophores encounter more xanthophores and fewer iridophores, participate in only a subset of potential interactions and fail to receive positional information necessary to terminate primary stripes or initiate secondary stripes. Interactions between xanthophores are hypothetical. ( c ) Pattern development in D. rerio. (1) Iridophores differentiate at the horizontal myoseptum. (2) Melanophores arise dispersed over the flank while iridophores express Csf1, which is also expressed in the skin. (3) Locally high levels of Csf1 promote xanthophore differentiation in the interstripe as interactions involving all three classes of pigment cells refine the pattern of stripes and interstripes and additional iridophores infiltrate the stripe. (4) Iridophores begin to emerge beyond the stripe and initiate a secondary interstripe. (5) Iridophores of the secondary interstripe terminate the primary stripe, promote differentiation of secondary interstripe xanthophores and specify the location of secondary stripe development. Adult xanthophore precursors, and, later, incompletely differentiated xanthophores are distributed sparsely in stripes as well [26] , [50] (not shown). ( d ) Pattern development in D. albolineatus . (1) Initially high expression of iridophore-independent Csf1 promotes early, widespread xanthophore development. (2) A few iridophores develop near the horizontal myoseptum posteriorly. (3) Melanophores begin to appear scattered over the flank as do additional iridophores. (4–5) Residual stripes begin to form posteriorly around the residual interstripe [35] , but this pattern is obscured by widespread melanophores and xanthophores that ultimately fail to resolve into stripes and interstripes. Full size image In D. rerio , these several interactions, combined with tissue-derived positional information and other factors, generate the body stripes and interstripes ( Fig. 5c ). Iridophores are the first adult pigment cells to differentiate [22] , [23] , [42] . Their precursors migrate from extra-hypodermal locations to the hypodermis where they differentiate, proliferate and organize in the vicinity of the horizontal myoseptum [47] , [48] , thereby establishing the primary interstripe ( Fig. 5c1 ). Melanophores are the second adult pigment cells to appear, and arise from highly motile precursors that also travel from extra-hypodermal locations, via peripheral nerves and other tissues, to reach the hypodermis [44] , [49] . Once in the hypodermis, these cells initiate their differentiation relatively widely over the flank [49] ( Fig. 5c2 ). Some newly differentiating melanophores—as well as persisting early larval melanophores—occur in the interstripe and migrate short distances to join the stripes; others initially in the interstripe die or are covered by iridophores [17] , [21] , [22] , [31] , [38] . Iridophores help to organize melanophores, and thereby specify the location and orientation of the primary stripes, and later colonize the primary stripe in smaller numbers (this study [22] , [23] ). Interstripe xanthophores are the last to appear ( Fig. 5c3 ) and develop from cells already in the hypodermis including embryonic xanthophores that transiently lose their pigment only to reacquire it later [26] . Xanthophore differentiation depends on TH as well as Csf1, which is supplied locally by iridophores and more globally by other cells in the skin [22] ; interactions between xanthophores and melanophores promote the segregation of these cell types into stripes and interstripes [19] , [20] , [26] , [28] ( Fig. 5c4 ). During later development interstripes and stripes are added. Our analyses of iridophore ablation phenotypes demonstrate an important role for iridophores in this process of pattern reiteration, specifically in terminating the primary melanophore stripe and specifying the position of the next, secondary melanophore stripe ( Fig. 5c6 ). These inferences and our observations of iridophore development (for example, Supplementary Movie 1 ) are consistent with a recent description of iridophore locations and clonal expansion [47] . Our study reveals very different events in D. albolineatus . In this species, pattern formation begins with an abundance of iridophore-independent Csf1, which promotes early, widespread xanthophore differentiation ( Fig. 5d1 ). Unlike primary interstripe iridophores in D. rerio , which impart positional information to melanophores [22] , [23] , the scattered population of xanthophores in D. albolineatus lacks positional information for melanophores. In addition, the primary interstripe is itself reduced and secondary interstripes do not form, possibly owing to repressive effects of xanthophores, although a definitive assessment of this idea requires additional analyses now underway. Thus, although D. albolineatus initiate interstripe and stripe development, especially posteriorly ( Fig. 5d2 ), and exhibit latent stripe-forming potential [31] , [35] , the combination of widespread xanthophores and an absence of secondary interstripe iridophores promotes a nearly uniform pattern of melanophores. We found that D. albolineatus express more Csf1 than D. rerio owing in part to cis regulatory changes at csf1a , and that enhanced Csf1 expression can drive the development of supernumerary xanthophores in D. rerio , resulting in the loss of stripes, similar to D. albolineatus. These findings also suggest excess Csf1 as a candidate mechanism allowing some xanthophores to differentiate in D. albolineatus even without TH [26] . Genetic analyses previously identified Csf1r or its pathway as potentially contributing to stripe loss in D. albolineatus and pattern alterations in other danios [9] , [31] : hybrids between D. albolineatus and wild-type D. rerio developed stripes, yet hybrids between D. albolineatus and xanthophore-deficient csf1r mutant D. rerio had disrupted stripes and xanthophores in a pattern resembling D. albolineatus . Our observations are consistent with a model in which excess Csf1 derived from D. albolineatus alleles, in conjunction with evolutionary changes affecting receptor–ligand interactions [31] , explain the disruption of stripes in hybrids between D. albolineatus and D. rerio mutant for csf1r . We have identified roles for Csf1 and differential xanthophore recruitment in the evolution of pattern differences between D. albolineatus and D. rerio . Yet, our findings do not exclude roles for additional factors, including changes to pigment cell autonomous interactions themselves, or other modifications to the tissue environment or hormonal milieu. Indeed, experiments with D. rerio did not recapitulate the smaller population of melanophores in D. albolineatus : in Csf1-overexpressing D. rerio , extra xanthophores were accompanied by extra melanophores, whereas in D. albolineatus , melanophores are fewer and more likely to die than in D. rerio [31] . This disparity may reflect species differences in the relative strengths of supportive and repressive interactions between melanophores and xanthophores [19] , [28] , [41] , as has also been suggested by genetic analyses [31] . Such possibilities are currently being investigated. In conclusion, our analyses demonstrate that changing the initial time and place at which pigment cells differentiate can result in ‘priority effects’ that alter subsequent pattern development. If pigment–cell autonomous interactions are an engine for pattern formation, our study illustrates that very different pattern outcomes can occur depending on the context in which this engine operates. Such considerations may help to explain the extraordinary diversification of pigment pattern in teleosts [8] , [11] , [51] , [52] and other ectothermic vertebrates [53] , [54] , [55] . Fish stocks, staging and rearing conditions D. rerio wild-type stock fish, WT(WA), were produced by crosses between the inbred genetic strains AB wp and wik or the progeny of these crosses. Iridophore-deficient bonaparte mutants are presumptive null alleles bnc2 utr16e1 (ref. 45 ). D. aff. albolineatus [31] stocks were obtained from tropical fish suppliers and have been inbred and maintained in the lab for more than eight generations. Transgenic lines were: Tg(hsp70l:csf1a-IRES-nlsCFP) wp.r.t4 ; Tg(hsp70l:kitlga) wp.r.t2 , Tg(csf1a rerio :mCherry) and Tg(csf1a alb :mCherry) in D. rerio ; Tg(csf1a rerio :mCherry ) and Tg(csf1a alb :mCherry) in D. albolineatus ; and TgBAC(foxd3:EGFP) n15 D. rerio (ref. 56 ), kindly provided by Alex Nechiporuk (Oregon Health Sciences University, Portland, OR, USA). Post-embryonic staging followed [42] . D. albolineatus reached each developmental stage at a larger size than D. rerio , so criteria such as fin ray development were used as an indicator of stage rather than standardized standard length. All fish stocks were reared in standard conditions of 14 h light:10 h dark at 28.5 °C, and fed Rotimac-fortified marine rotifers followed by brine shrimp and flake food. For transgene inductions of Tg(hsp70l:csf1a-IRES-nlsCFP) wp.r.t4 and Tg(hsp70l:kitlga) wp.r.t2 , fish were heat-shocked at 38 °C twice daily for 1 h through adult pigment pattern formation. All experiments were conducted with approval of the University of Washington Animal Care and Use Committee and complied with United States federal guidelines for ethical use of animals in research. Transgene construction and microinjection To generate csf1a reporter lines, we cloned ~9 kb proximal to the csf1a start site from both species into a 5′ Gateway vector. Transgenes were then assembled by Gateway cloning of entry plasmids into pDestTol2CG2 containing Tol2 repeats for efficient genomic integration and cmlc2:EGFP as a transgenesis marker [57] , [58] . Microinjection of plasmids and Tol2 messenger RNA followed standard methods. Progeny of F0 injected fish were screened for cmlc2 :EGFP and used to establish independent, stable transgenic lines in D. rerio ( Tg(csf1a rerio9.1 :mCherry) , n =8; Tg(csf1a alb9.2 :mCherry) , n =3); ( Tg(csf1a rerio9.1Δ338 :mCherry) , n =3; Tg(csf1a rerio9.1Δ1039 :mCherry) , n =6) and D. albolineatus ( Tg(csf1a rerio9.1 :mCherry) , n =1; Tg(csf1a alb9.2 :mCherry) , n =3)). Conservation and divergence of csf1a regulatory regions was evaluated using the UCSC Genome Browser [59] . Ablation of secondary interstripe iridophores in larvae mosaic for pnp4a:nVenus-2a-nfnB followed ref. 22 , with Mtz treatment beginning at stage PR. RT-PCR and quantitative RT-PCR For quantitative RT-PCR in D. rerio and D. albolineatus , skins and underlying tissue were collected from AR+, DR+, PB+ and J stage larvae. To generate interspecific hybrids for quantitative RT-PCR, a D. rerio female was crossed to a D. albolineatus male by in vitro fertilization and resulting larvae were collected at AR+. All tissues were placed directly into either Trizol Reagent (Invitrogen) or RNAlater (Ambion). RNA was isolated using either the RNaqueous Microkit (Ambion) or Trizol, followed by LiCl precipitation. Complementary DNA (cDNA) was synthesized using the iScript cDNA Synthesis Kit (Bio-Rad). Quantitative RT-PCRs were performed and analysed on a StepOnePlus System (Life Technologies) using Custom Taqman Gene Expression Assays, designed to bind either conserved sites ( csf1a , csf1b and rpl13a ) or species-specific sites ( csf1a hybrid analysis), and Taqman Gene Expression Master Mix (Life Technologies). For assays of expression from species-specific alleles in hybrids, abundances estimated from probes specific to each allele were normalized to a common probe recognizing both alleles. All assays were replicated across ≥3 biological samples, each having three technical replicates. To detect mCherry transcripts in D. rerio Tg(csf1a rerio9.1 :mCherry) and Tg(csf1a alb9.2 :mCherry) transgenic lines, individual larvae were collected at stage PR. Heads and tails were removed and trunks were placed in RNAlater (Ambion). RNA was isolated using the Direct-zol RNA Kit (Zymo Research, R2050) and cDNA synthesized using the iScript cDNA Synthesis Kit (Bio-Rad). For RT-PCR of isolated iridophores, late metamorphic/early juvenile larvae were euthanized and skins were collected in phosphate-buffered saline (PBS). Skins were vortexed briefly to remove scales, then centrifuged gently and washed again in PBS. Tissue was incubated 10 min at 37 °C in 0.25% trypsin-EDTA (Invitrogen). Trypsin was removed and the tissue was incubated for 10 min at 37 °C in tyrpsin-inhibitor (Sigma T6414) with 3 mg ml −1 collagenase, and 2 μl Dnase I, RNase-Free (Thermo Scientific), followed by gentle pipetting until skins were completely dissociated. Cells were then washed in PBS and filtered through a 40-μm cell strainer. Cell were placed on a glass-bottom dish and examined on a Zeiss Observer inverted compound microscope. A minimum of 50 iridophores were picked using a Narishige 1M 9B microinjector, expelled into PBS, then repicked and expelled directly into Resuspension Buffer. cDNA was synthesized using Superscript III Cells Direct cDNA Synthesis Kit (Invitrogen). RT-PCR was performed with the following primer sets (forward, reverse): actb1, 5′- ACTGGGATGACATGGAGAAGAT -3′, 5′- GTGTTGAAGGTCTCGAACATGA -3′; csf1a, 5′- CAACAACTGAGCCAACACATAAATA -3′, 5′- GGGATCTGTGGTCTTTGCTGAT -3′; csf1b, 5′- AACACCCCTGTTAACTGGACCT -3′, 5′- GAGGCAGTAGGCAGTGAGAAGA -3′; mdkb, 5′- TGGACACTTTAATGGTGGTCTG -3′; mCherry, 5′- CCAGCTTGATGTTGACGTTG -3′, 5′- AGGACGGCGAGTTCATCTAC -3′; pnp4a, 5′- GAAAAGTTTGGTCCACGATTTC -3′, 5′- TACTCATTCCAACTGCATCCAC -3′. Immunohistochemistry For immunohistochemistry, fish were fixed in 4% paraformaldehyde for 30 min at room temperature, washed with PBS, transferred to 15% sucrose, followed by 30% sucrose and then embedded and frozen in OCT media. Cryosections of 20 μm thickness were collected on Microfrost Plus slides (Fisher) and allowed to dry. Slides were washed in PBS and then fixed in 4% paraformaldehyde for 10 min at room temperature followed by additional PBS washes. Sections were blocked in PBS containing 5% heat-inactivated goat serum and 0.1% Triton-X, then incubated overnight at 4 °C with primary antibody. Antibodies were monoclonal rat anti-mCherry (1:300; Life Technologies, M11217), and polyclonal rabbit anti-Human BNC2 antibody (1:350). After washes, slides were incubated with secondary antibodies (Alexa Fluor 488, 568), washed in PBS and imaged on a Zeiss Observer inverted microscope equipped with Yokogawa CSU-X1M5000 laser spinning disk. Imaging and quantitative analysis Fish were imaged on an Olympus SZX-12 stereomicroscope, Zeiss Axioplan 2i compound microscope or Zeiss Observer inverted compound microscope using Zeiss Axiocam HR or MRc cameras, or a Photometrics Evolve EMCCD camera and Axiovision software. Images were colour balanced and in some instances processed to facilitate visualization of xanthophores in Adobe Photoshop; comparable sets of images across genetic backgrounds or treatments were processed identically. For repeated imaging of individuals, fish were reared separately in glass beakers, then immediately prior to imaging were treated with 10 mM epinephrine to contract pigment granules towards cell centres, then anesthetized briefly, imaged and allowed to recover. Resulting images were re-scaled and aligned in Photoshop then exported as animated movies. To quantify melanophore dorsal–ventral positions, we measured the distance of each melanophore to the dorsal and ventral margins of the myotome and divided dorsal length by the total distance. For pnp4a:nVenus-2a-nfnB mosaic iridophore ablations and controls, positions were determined for all melanophores ventral to the horizontal myoseptum, in the area bordered by the anterior and posterior ends of the anal fin. For D. albolineatus , wild-type D. rerio , bnc2 mutant D. rerio and Tg(hsp70l:csf1a-IRES-nlsCFP) wp.r.t4 , melanophore positions were assessed for all melanophores ventral to the horizontal myoseptum, in the anterior third of the area between the anterior and posterior ends of the anal fin. To assess segregation versus intermingling of melanophores and xanthophore k-nearest-neighbour classifications were conducted using a MATLAB routine written in-house (MATLAB R2011a, Mathworks, Natick, MA, USA). For each fish, an average of the five nearest-neighbour distances were calculated for each cell from images taken at the border of the ventral melanophore stripe and the secondary ventral iridophore stripe or this region in individuals that did develop iridophores. Melanophore–xanthophore structure indices shown are the ratios of mean melanophore–xanthophore nearest-neighbour distances relative to the melanophore–melanophore nearest-neighbour distance. Other metrics for describing spatial segregation from nearest-neighbour values yielded equivalent results. Analyses of total melanophore numbers and melanophore–xanthophore segregation used ln -transformed-dependent values to correct for heteroscedasticity of residuals. All statistical analyses were performed using JMP 8.0.2 (SAS Institute, Cary, NC). How to cite this article : Patterson L. B., et al . Pigment cell interactions and differential xanthophore recruitment underlying zebrafish stripe reiteration and Danio pattern evolution. Nat. Commun. 5:5299 doi: 10.1038/ncomms6299 (2014).